Natural variation inPTB1regulates rice seed setting rate by controlling pollen tube growth Grain number, panicle seed setting rate, panicle number and grain weight are the most important components of rice grain yield. To date, several genes related to grain weight, grain number and panicle number have been described in rice. However, no genes regulating the panicle seed setting rate have been functionally characterized. Here we show that the domestication-related POLLEN TUBE BLOCKED 1 ( PTB1 ), a RING-type E3 ubiquitin ligase, positively regulates the rice panicle seed setting rate by promoting pollen tube growth. The natural variation in expression of PTB1 which is affected by the promoter haplotype and the environmental temperature, correlates with the rice panicle seed setting rate. Our results support the hypothesis that PTB1 is an important maternal sporophytic factor of pollen tube growth and a key modulator of the rice panicle seed setting rate. This finding has implications for the improvement of rice yield. Rice ( Oryza sativa L.) is one of the most important food crops because it is the main staple food for more than half of the world’s population. Grain weight, grain number, panicle number and panicle seed setting rate (PSSR) are the main determinants of rice grain yield. To date, several genes related to grain yield have been identified and functionally characterized. Among these genes, GS3 (refs 1 , 2 ), GS5 (ref. 3 ), GW2 (ref. 4 ), qSW5 (ref. 5 ) (also known as GW5 (ref. 6 )), GW8 (ref. 7 ), GL3.1 (ref. 8 ) and TGW6 (ref. 9 ) are involved in grain weight or size regulation and Gn1a (ref. 10 ) is associated with panicle grain number. Moreover, GIF1 (ref. 11 ) is crucial for seed filling, Ghd7 (ref. 12 ) regulates the growth period and DEP1 (ref. 13 ) and IPA1 (ref. 14 ) (also known as WFP (ref. 15 )) are involved in plant architecture construction. However, to our knowledge, no genes regulating PSSR, one of the most important yield determinants, have been functionally characterized. In addition, rice PSSR is susceptible to environmental conditions, which often lead to large rice yield losses and threatens the safety of rice production. Additionally, PSSR has become a bottleneck that limits the further improvement of rice grain yield via the use of heterosis because many hybrid rice varieties exhibit sharp decreases in PSSR compared with their parents. Therefore, disclosure of the molecular mechanism underlying PSSR regulation and its immediate implications are needed for the improvement of rice production. As the female gametes are deeply imbedded in the maternal tissues of the ovary, flowering plants generate a unique system, the pollen tube (PT), to accomplish the goal of reproduction [16] . In rice, pollen grains induce the formation of the PTs after germination on the stigma and begin the long journey to deliver the sperm cells. The PTs then enter the stigma and grow toward and through the style transmission tract (STT) to reach the micropyle of the embryo sac. Finally, the PTs arrive at the female gametophyte and release the sperm cell contents for double fertilization. The mechanism that precisely directs the long navigation of the PT from the stigma toward the female gametophyte has been the subject of investigation for several decades. It is now widely accepted that PTs receive multiple, stage-specific guidance cues during this long and arduous process [16] . Before entering the ovary, PT guidance requires abundant communication with the surrounding sporophytic maternal tissues; however, after reaching the micropyle of the embryo sac, PT guidance is thought to be primarily under gametophytic control. Various candidates for PT attractants have been reported, including the lily small cell wall protein chemocyanin [17] and the water gradient in lipids [18] , for directional growth of PTs at the stigma. γ-aminobutyric acid (GABA), controlled by the Arabidopsis POP2 gene [19] , has been suggested as a sporophytic signal for STT growth and ovule targeting. ZmEA1 (ref. 20 ) has been demonstrated as a candidate for PT guidance derived from the maize synergid cell. Additionally, recent work has characterized two CRP-type PT attractants, LURE1 and LURE2 (ref. 21 ), from the synergid cell of Torenia fournieri . However, unlike the factors guiding PTs, the maternal sporophytic factors regulating PT growth in the STT remain largely unknown; few of these factors, such as lily SCAs [22] , which are involved in the adhesion of PTs to the STT, and Nicotiana TTS [23] , [24] , which is necessary for PT growth in the STT, have been elucidated. Especially in rice, a model monocotyledonous plant and the most important agricultural plant, the regulation of PT growth by the maternal parent is not well understood. Here we report that POLLEN TUBE BLOCKED 1 ( PTB1 ) positively regulates rice PSSR by controlling PT growth. The female sterile mutant ptb1 is normal in terms of the female apparatus; however, PT growth is blocked soon after entering the STT. The PTB1 gene, which encodes a RING-type E3 ubiquitin ligase, promotes PT growth by controlling the amount and depth of growth of PTs in the rice reproductive tract. The PTB1 expression level significantly correlates with rice PSSR both in transgenic plants and in natural populations, resulting in a major modulation of rice PSSR. We also show that the PTB1 locus was selected by ancient humans during rice domestication and that the haplotype of the promoter has a role in determining the expression level of PTB1 . Our data therefore reveal a key maternal sporophytic factor for PT growth and an important positive regulator of rice PSSR. Identification of a low-PSSR mutant in rice We discovered a rice mutant with an extremely low PSSR (1.80±0.140%, Fig. 1a–d ) while screening for fertility mutations. The mutant exhibits no obvious difference from the wild type (WT) except a sterile phenotype. The floret structure and pollen fertility are equal to those of the WT ( Fig. 1e–h ). Reciprocal crossing with several rice lines showed that when the mutant was crossed as a pollen donor, the seeds set normally; however, when used as a pollen receiver, no seeds were obtained. This finding demonstrates that the low PSSR of the mutant was due to female-specific sterility ( Supplementary Table S1 ). Genetic analysis within several populations indicated that the mutation was controlled by a single recessive gene ( Supplementary Table S2 ). 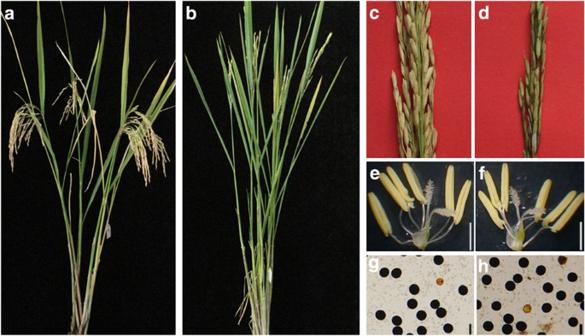Figure 1: Phenotypic comparisons of the WT and mutant plants. (a) Plant phenotype of the WT. (b) Plant phenotype of the mutant. (c) Panicle of the WT. (d) Panicle of the mutant. (e) Floral structure of the WT. (f) Floral structure of the mutant. Scale bars, 1 mm. (g) I2-KI staining of pollen grains in the WT. (h) I2-KI staining of pollen grains in the mutant. Scale bars, 50 μm. Figure 1: Phenotypic comparisons of the WT and mutant plants. ( a ) Plant phenotype of the WT. ( b ) Plant phenotype of the mutant. ( c ) Panicle of the WT. ( d ) Panicle of the mutant. ( e ) Floral structure of the WT. ( f ) Floral structure of the mutant. Scale bars, 1 mm. ( g ) I 2 -KI staining of pollen grains in the WT. ( h ) I 2 -KI staining of pollen grains in the mutant. Scale bars, 50 μm. Full size image To clarify the sterile causation, mature embryo sacs were examined using a whole-mount eosin B staining confocal laser scanning microscopy (WE-CLSM) method [25] . The results showed that almost all of the mutant mature embryo sacs were of the typical Polygonum type and had complete inner components with apparent polarity ( Supplementary Fig. S1 ), suggesting that the mature embryo sacs of the mutant are functional and that the low PSSR of the mutant may result from a defect in the pollination process. PT growth is blocked in the mutant STT To further investigate the behaviour of PT growth, we collected a large amount of self-pollinated pistils for fluorescence microscopic observations. Pollen grains became attached to the stigmas and generated PT at 5 min after pollination (AP) ( Fig. 2a,b ). PTs then entered the stigmas and grew rapidly at 10 min AP ( Fig. 2c,d ). At these two stages, no significant differences were detected between the mutant and WT. However, PT growth diverged at 20 min AP. PTs in the WT plants easily entered the STT and grew rapidly ( Fig. 2e ), whereas PTs in the mutants appeared to experience difficulty in entering the STT and were detained in the lower end of the stigma ( Fig. 2f ). In the WT, several PTs reached the ovary, the base ovule and the micropyle at 30, 45 and 60 min AP, respectively; however, PTs in the mutant were abnormally blocked in the STT ( Fig. 2g–l ). Consequently, no PTs were found entering the embryo sac in the mutant, even at 2–48 h AP ( Fig. 2m–o ). Simultaneously, PTs in the mutant exhibited more obvious tip defects than PTs in the WT ( Fig. 2p–t ). Interestingly, intense callose deposition was observed on the ovule surface in the mutant; this deposition was absent in the WT ( Fig. 2m,n ). These characteristics were similar to those observed in a previously examined mutant [26] except for the callose deposition and the pistil anatomical structure. Therefore, the female sterility of the mutant resulted from the blocking of PT growth in the stigma and the STT, and the mutant was named pollen tube blocked 1(ptb1) . 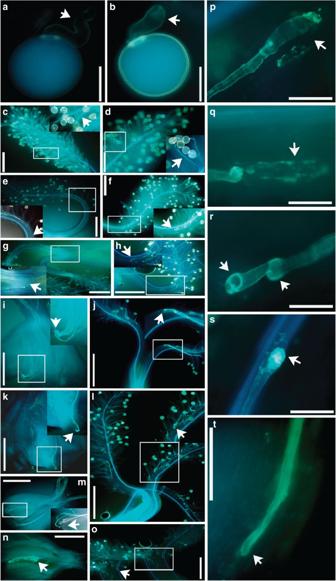Figure 2: PT growth observations ofptb1. (a) PT growth in the WT, 5 min AP. (b) PT growth inptb1, 5 min AP. (c) PT growth in the WT, 10 min AP. (d) PT growth inptb1, 10 min AP. (e) PT growth in the WT, 20 min AP. (f) PT growth inptb1, 20 min AP. (g) PT growth in the WT, 30 min AP. (h) PT growth inptb1, 30 min AP. (i) PT growth in the WT, 45 min AP. (j) PT growth inptb1, 45 min AP. (k) PT growth in the WT, 60 min AP. (l) PT growth inptb1, 60 min AP. (m) PT growth in the WT, 120 min AP. (n) PT growth inptb1, 120 min AP. (o) PT growth inptb1, 120 min AP. (p) A broken pollen tip. (q) A diffused pollen tip. (r) A distorted and branched pollen tip. (s) An agglomerated pollen tip. (t) A normal pollen tip in the WT. Callose deposition on the surface of the ovule ofptb1(n), which is not present in the WT (k,m). The region boxed with a white line is magnified in another window in the same panel. An arrow indicates the germinated PT (a–d), the PT tip (e–m,o,t) or the noted abnormalities (n,p–s). More than 30 samples for each time-point were collected and observed. Scale bars, 50 μm in (a,b,p–t); 300 μm in (c–o). Figure 2: PT growth observations of ptb1 . ( a ) PT growth in the WT, 5 min AP. ( b ) PT growth in ptb1 , 5 min AP. ( c ) PT growth in the WT, 10 min AP. ( d ) PT growth in ptb1 , 10 min AP. ( e ) PT growth in the WT, 20 min AP. ( f ) PT growth in ptb1 , 20 min AP. ( g ) PT growth in the WT, 30 min AP. ( h ) PT growth in ptb1 , 30 min AP. ( i ) PT growth in the WT, 45 min AP. ( j ) PT growth in ptb1 , 45 min AP. ( k ) PT growth in the WT, 60 min AP. ( l ) PT growth in ptb1 , 60 min AP. ( m ) PT growth in the WT, 120 min AP. ( n ) PT growth in ptb1 , 120 min AP. ( o ) PT growth in ptb1 , 120 min AP. ( p ) A broken pollen tip. ( q ) A diffused pollen tip. ( r ) A distorted and branched pollen tip. ( s ) An agglomerated pollen tip. ( t ) A normal pollen tip in the WT. Callose deposition on the surface of the ovule of ptb1 ( n ), which is not present in the WT ( k , m ). The region boxed with a white line is magnified in another window in the same panel. An arrow indicates the germinated PT ( a – d ), the PT tip ( e – m , o , t ) or the noted abnormalities ( n , p – s ). More than 30 samples for each time-point were collected and observed. Scale bars, 50 μm in ( a , b , p – t ); 300 μm in ( c – o ). Full size image We also surveyed PT growth in the STT of several controlled pollinated reciprocal crosses. When the mutant was crossed as a pollen donor with other WT lines, PTs grew quite normally and easily reached the micropyle for fertilization ( Fig. 3a,b ). However, when the mutant stigmas were sprinkled with normal foreign pollen grains, we observed the same abnormalities as those seen in the self-pollinated mutant pistils ( Fig. 3c–f ). These results, together with those obtained during investigations of pollen fertility in the mutant ( Fig. 1g,h ) and the panicle seed setting of reciprocal crossing ( Supplementary Table S1 ), demonstrate that the PT growth arrest of the mutant is caused by a maternal defect and that the mutation does not affect the function of the male gametophyte. 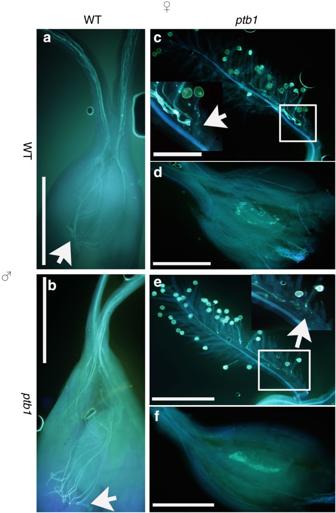Figure 3: PT growth observations of the reciprocal crossing. (a) PT growth within pistils of the cross WT(♀) × WT(♂). (b) PT growth within pistils of the cross WT(♀) ×ptb1(♂). (c) PT growth within pistil styles of the crossptb1(♀) × WT(♂). (d) PT growth within the ovary of the crossptb1(♀) × WT(♂). (e) PT growth within pistil styles of the crossptb1(♀) ×ptb1(♂). (f) PT growth within the ovary of the crossptb1(♀) ×ptb1(♂). ♂, crossed as male parents; ♀, crossed as female parents. Arrows indicate the PT tip. Samples for fluorescence microscopic observation were collected at 2 h AP,n>30. Scale bars, 400 μm. Figure 3: PT growth observations of the reciprocal crossing. ( a ) PT growth within pistils of the cross WT(♀) × WT(♂). ( b ) PT growth within pistils of the cross WT(♀) × ptb1 (♂). ( c ) PT growth within pistil styles of the cross ptb1 (♀) × WT(♂). ( d ) PT growth within the ovary of the cross ptb1 (♀) × WT(♂). ( e ) PT growth within pistil styles of the cross ptb1 (♀) × ptb1 (♂). ( f ) PT growth within the ovary of the cross ptb1 (♀) × ptb1 (♂). ♂, crossed as male parents; ♀, crossed as female parents. Arrows indicate the PT tip. Samples for fluorescence microscopic observation were collected at 2 h AP, n >30. Scale bars, 400 μm. Full size image We further observed the anatomical structure and extracellular matrix (ECM) components of the female reproductive tract using previously reported methods [25] , [27] . The results showed that the overall cellular structure of the STT in ptb1 was comparable to that in the WT ( Supplementary Fig. S2a–d ). Moreover, a similar degree of Alcian blue staining was detected in ptb1 and WT STT ( Supplementary Fig. S2e–l ), suggesting that the ECM in ptb1 was normal and that the overall composition was not different from that in the WT. We thus infer that the arrest of the PT growth in ptb1 is not caused by a structural defect in the female reproductive tract. Map-based cloning of PTB1 By employing a map-based clone strategy in a large F 2 population of ptb1 /Gui630, the PTB1 gene was localized to a 72-kb physical region on rice chromosome 5, which contains nine predicted genes in total ( Fig. 4a–d ). Comparative sequencing of the entire region revealed a 470-nt deletion in the coding region of the LOC_Os05g05280 gene in ptb1 ( Fig. 4e ) that causes a 232-nt mRNA deletion, resulting in the occurrence of a premature termination codon in its predicted open reading frame ( Supplementary Fig. S3 ). The corresponding deletions were also confirmed by PCR or RT–PCR analysis in the sterile F 2 plants ( Fig. 4f,g ), suggesting that the deletion in the LOC_Os05g05280 gene might cause the abnormal PT growth in ptb1 . 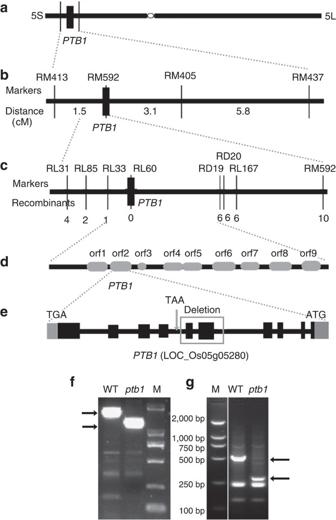Figure 4: Positional cloning ofPTB1. (a)PTB1was first mapped to the short arm of chromosome 5 using a bulked segregation analysis. (b)PTB1was then delimited to a genetic region flanked with the markers RM413 and RM405 and co-segregated with RM592 in a small population (n=100). (c)PTB1was finally narrowed down to a 72-kb region between markers RL33 and RD19 and co-segregated with Rl60 in a large population (n=2,382). (d) In total, nine genes were predicted within the 72-kb region. (e) Sequencing revealed a 470-nt deletion in the coding region of the mutant LOC_Os05g05280 gene; this deletion resulted in a premature termination of the predicted open reading frame. (f) PCR confirmation of the corresponding deletions (arrowed) in some F2sterile plants (n>50). (g) RT–PCR confirmation of the corresponding deletions (arrowed) in some F2sterile plants (n>50). Figure 4: Positional cloning of PTB1 . ( a ) PTB1 was first mapped to the short arm of chromosome 5 using a bulked segregation analysis. ( b ) PTB1 was then delimited to a genetic region flanked with the markers RM413 and RM405 and co-segregated with RM592 in a small population ( n =100). ( c ) PTB1 was finally narrowed down to a 72-kb region between markers RL33 and RD19 and co-segregated with Rl60 in a large population ( n =2,382). ( d ) In total, nine genes were predicted within the 72-kb region. ( e ) Sequencing revealed a 470-nt deletion in the coding region of the mutant LOC_Os05g05280 gene; this deletion resulted in a premature termination of the predicted open reading frame. ( f ) PCR confirmation of the corresponding deletions (arrowed) in some F 2 sterile plants ( n >50). ( g ) RT–PCR confirmation of the corresponding deletions (arrowed) in some F 2 sterile plants ( n >50). Full size image To determine whether LOC_Os05g05280 underlies the PTB1 gene, we generated a construct by placing a ~2.66-kb DNA fragment containing a ~1.5-kb native promoter and an ~1.16-kb full-length cDNA of LOC_Os05g05280 into vector pHB [28] . As the mutant was sterile and could not generate seeds for callus induction, we introduced this construct into the young panicle-originated callus of the ptb1 mutant by Agrobacterium -mediated transformation. All of the resulting transgenic plants rescued the sterility phenotype ( Fig. 5a–d ), although the PSSR varied ( Supplementary Table S3 ). We also examined all T 1 families from T 0 plants and observed perfect co-segregation between the transgene and the rescued phenotype ( Fig. 5e ). Therefore, we conclude that LOC_Os05g05280 is the gene responsible for PTB1 . 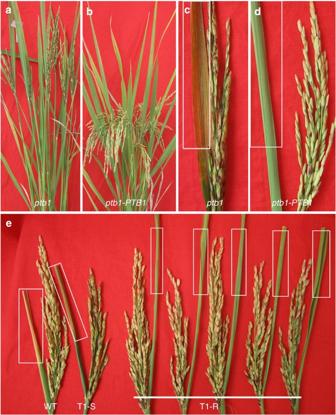Figure 5: Functional complementation ofptb1. (a) Plant phenotype ofptb1. (b) Plant phenotype of thePTB1-transformedptb1plants (ptb1–PTB1). (c) Panicle phenotype ofptb1. (d) Panicle phenotype of theptb1–PTB1transgenic plants. (e) Co-segregation of the introducedPTB1and the fertile panicle phenotype. The white lined box indicates that the transgenic plants were resistant to the herbicide Barstar (a Barstar resistance gene was placed in the T-DNA region of the pHB vector) and non-transformed plants remained sensitive. T1-S, Barstar-sensitive T1plants; T1-R, Barstar-resistant T1plants. Figure 5: Functional complementation of ptb1 . ( a ) Plant phenotype of ptb1 . ( b ) Plant phenotype of the PTB1 -transformed ptb1 plants ( ptb1–PTB1 ). ( c ) Panicle phenotype of ptb1 . ( d ) Panicle phenotype of the ptb1–PTB1 transgenic plants. ( e ) Co-segregation of the introduced PTB1 and the fertile panicle phenotype. The white lined box indicates that the transgenic plants were resistant to the herbicide Barstar (a Barstar resistance gene was placed in the T-DNA region of the pHB vector) and non-transformed plants remained sensitive. T 1 -S, Barstar-sensitive T 1 plants; T 1 -R, Barstar-resistant T 1 plants. Full size image PTB1 positively regulates rice PSSR by controlling PT growth We generated several transgenic plants with large PSSR variations in a ptb1 background ( Supplementary Table S3 ). We first divided these plants into three categories according to their PSSRs ( Fig. 6a ). Investigations of the PT growth revealed fundamental differences among these categories ( Fig. 6b ). In the lower group, although PT growth was apparently deeper than in the ptb1 mutant, growth always ceased sharply at the sporophytic STT nearing the chalazal end of the embryo sac. In the moderate group, more PTs reached the chalazal end of the embryo sac, and a limited number of PTs continued their journey to reach the micropyle. However, in the higher group, many PTs continued past the chalazal end of the embryo sac and easily reached the micropyle for further fertilization. These results demonstrated that the PSSR in the transgenic plants was directly determined by the amount and growth depth of the PTs ( Fig. 6a,b ). 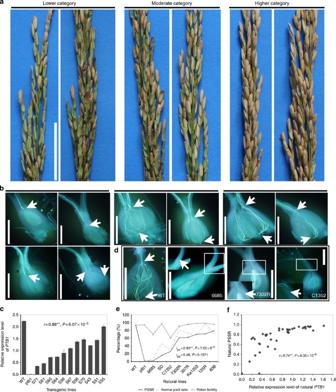Figure 6:PTB1affects rice PSSR by controlling PT growth. (a) Panicle phenotype of each category, as defined by PSSR (lower category, PSSR⩽30%; moderate category, 30%⩽PSSR⩽70%; higher category, PSSR⩾70%). (b) PT growth in each category (from left to right, lower, moderate and higher categories). Arrows indicate the chalazal end of the embryo sac and the micropyle. (c) The correlation between PSSR and the expression level of introducedPTB1. Data are given as mean±s.e.m. (n=3). PSSRs are listed inSupplementary Table S3. (d) PT growth abnormalities observed in several lines with lower PSSR. The region boxed using a white line is shown magnified in another window in the same panel. Arrows indicate the chalazal end of the embryo sac and the micropyle (in WT) and the PT tip (in 6685, 7302R and C1352). (e) Determinants of natural PSSR variations. PSSR and pollen fertility are presented as the mean±s.e.m. (n=3), and the normal pistil ratio was calculated by comparing the ratio of the PT-normal-grown pistils to the total of individuals observed using fluorescence microscopy (n>30).rpp, the correlation between PSSR and pollen fertility;rpn, the correlation between PSSR and normal pistil ratio. (f) The correlation between natural PSSR and the expression level of nativePTB1in a natural population. Allrvalues are based on two-tailed Pearson correlation analyses. Samples for fluorescence microscopic observation were collected at 2 h AP,n>30. Scale bars, 5 cm in (a) and 400 μm in (b) and (d). Figure 6: PTB1 affects rice PSSR by controlling PT growth. ( a ) Panicle phenotype of each category, as defined by PSSR (lower category, PSSR ⩽ 30%; moderate category, 30% ⩽ PSSR ⩽ 70%; higher category, PSSR ⩾ 70%). ( b ) PT growth in each category (from left to right, lower, moderate and higher categories). Arrows indicate the chalazal end of the embryo sac and the micropyle. ( c ) The correlation between PSSR and the expression level of introduced PTB1 . Data are given as mean±s.e.m. ( n =3). PSSRs are listed in Supplementary Table S3 . ( d ) PT growth abnormalities observed in several lines with lower PSSR. The region boxed using a white line is shown magnified in another window in the same panel. Arrows indicate the chalazal end of the embryo sac and the micropyle (in WT) and the PT tip (in 6685, 7302R and C1352). ( e ) Determinants of natural PSSR variations. PSSR and pollen fertility are presented as the mean±s.e.m. ( n =3), and the normal pistil ratio was calculated by comparing the ratio of the PT-normal-grown pistils to the total of individuals observed using fluorescence microscopy ( n >30). r pp , the correlation between PSSR and pollen fertility; r pn , the correlation between PSSR and normal pistil ratio. ( f ) The correlation between natural PSSR and the expression level of native PTB1 in a natural population. All r values are based on two-tailed Pearson correlation analyses. Samples for fluorescence microscopic observation were collected at 2 h AP, n >30. Scale bars, 5 cm in ( a ) and 400 μm in ( b ) and ( d ). Full size image To test whether the PT growth behaviour was caused by the different expression level of the introduced PTB1 , we determined the expression level among those independent transgenic lines. q-PCR experiments demonstrated that the PSSR significantly correlated with the expression level of the introduced PTB1 in the ptb1 background ( Fig. 6c and Supplementary Table S3 , r =0.88, P <0.01, Pearson correlation analysis). We thus concluded that PTB1 has a key role in regulating the amount and depth of PT growth in the rice reproductive tract, and consequently determined the PSSR in a ptb1 background. The dosage effect of PTB1 also suggested a positive regulation of PTB1 on rice PSSR. We then investigated whether PTB1 works universally in natural populations. We first inspected the factors involved in lower PSSRs within several rice plants that exhibited panicle fertility defects. Although pollen fertilities declined in some lines, PT growth in almost all lines was obviously affected, and the abnormalities were quite similar to those observed in the mutant background ( Fig. 6d,e ). A significant correlation between PSSR and PT growth (quantified as the normal pistil ratio) was detected ( Fig. 6e , r =0.93, P <0.01, Pearson correlation analysis). This finding suggests that PT growth in the style had a greater influence on rice PSSR than pollen fertility and that this might be the major determinant of the natural variation of rice PSSR. We next tracked natural PTB1 transcript levels within a panel of >40 rice varieties, representing a wide range of variation in PSSR ( Supplementary Table S4 ). Generally, the results showed that higher or lower PSSRs were always accompanied by higher or lower expression levels of natural PTB1 , respectively, resulting in a significant correlation between PSSR and PTB1 expression among the natural population ( Fig. 6f and Supplementary Table S4 , r =0.74, P <0.01, Pearson correlation analysis). In addition, an independent dwarf mutant, c1352, exhibited a drastic decrease in PSSR ( Supplementary Fig. S4a , P <0.01, t -test) and obvious PT growth arrests in the STT ( Fig. 6d ), and was accompanied by significant decreases in PTB1 expression ( Supplementary Fig. S4b , P <0.01, t -test). Together, these data indicated that PTB1 controlled rice PSSR universally and that variations in its expression largely determined the final PSSR. As PSSR was positively affected by PTB1 , we then tested its potential for improving rice PSSR. A pHB construct, in which the PTB1 gene was driven by the 2 × 35S promoter, was introduced into kasalath. Investigation indicated an apparent increase in the PSSR of the transgenic plants ( Supplementary Fig. S5a , P <0.01, t -test). The increased PSSR was further confirmed to be a consequence of PTB1 overexpression based on q-PCR analysis ( Supplementary Fig. S5b , P <0.01, t -test). These results further confirmed the influence of PTB1 expression on PSSR regulation and indicated the potential of PTB1 for use in rice yield improvement. PTB1 is a domestication-related gene We next sequenced the PTB1 promoter and the full-length coding sequence region in a total of 107 rice accessions, including 42 indica cultivars, 44 japonica cultivars and 21 O. rufipogon accessions ( Supplementary Data 1 ). Twenty-three variation sites within the promoter region and 14 sites within the coding sequence region were totally identified, of which five caused amino-acid substitutions. Sequence variation analysis completely identified 16 haplotypes in O. rufipogon ; however, only three haplotypes (types 1, 12 and 16) were present in O. sativa. This finding might suggest that the PTB1 locus was selected by ancient humans during rice domestication ( Fig. 7a,b ). A population investigation revealed a clear bias for both sub-species of O. sativa : ~98% of indica rice cultivars were in haplotypes of Type 12 or 16 (two highly similar types with few SNPs within the promoter), whereas ~75% of japonica rice cultivars were in the substantially distinct Type 1, suggesting that PTB1 was an indica – japonica -differentiated gene ( Fig. 7a,b , Supplementary Data 1 ). The limited number of prevalent haplotypes in indica rice also implied strong selection during rice domestication. Indeed, a recent large-scale, genome-wide analysis identified a selective sweep region around the PTB1 gene within the indica population [29] . 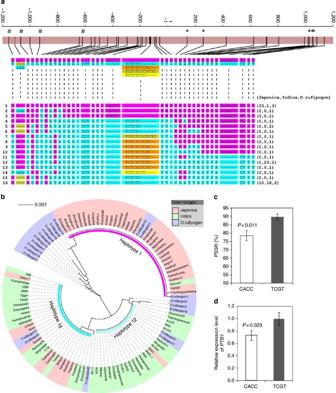Figure 7: Haplotype analysis of the promoter and coding sequence ofPTB1. (a) Distribution of DNA polymorphisms within thePTB1promoter and the coding sequence region and the resulting haplotypes identified among full populations. Different background colours indicate different nucleotides withnipponbare. Numbers in brackets indicate, in turn, the individual number ofjaponica,indicaandO. rufipogonaccessions that corresponded to the given haplotype. *Represents an amino acid substitution and#indicates the causal SNP of the promoter. (b) Phylogenetic tree of the full population calculated from 37 polymorphic sites ofPTB1. Two major groups, thejaponicagroup (haplotype 1) and theindicagroup (haplotypes 12 and 16), were identified inO. sativa. (c) Association of haplotypes with PSSR. (d) Association ofPTB1haplotypes withPTB1expression level. Values represent the mean±s.e.m. of at least two biological samples. AllP-values are based on one-tailedt-tests of corresponding data fromSupplementary Data 1. Figure 7: Haplotype analysis of the promoter and coding sequence of PTB1 . ( a ) Distribution of DNA polymorphisms within the PTB1 promoter and the coding sequence region and the resulting haplotypes identified among full populations. Different background colours indicate different nucleotides with nipponbare . Numbers in brackets indicate, in turn, the individual number of japonica , indica and O. rufipogon accessions that corresponded to the given haplotype. *Represents an amino acid substitution and # indicates the causal SNP of the promoter. ( b ) Phylogenetic tree of the full population calculated from 37 polymorphic sites of PTB1 . Two major groups, the japonica group (haplotype 1) and the indica group (haplotypes 12 and 16), were identified in O. sativa . ( c ) Association of haplotypes with PSSR. ( d ) Association of PTB1 haplotypes with PTB1 expression level. Values represent the mean±s.e.m. of at least two biological samples. All P -values are based on one-tailed t -tests of corresponding data from Supplementary Data 1 . Full size image We further investigated the possible role of allelic variation within the PTB1 promoter. The results of association tests suggested that two haplotypes (CACC and TCGT), which were determined by four SNPs (−1,156, −1,069, −931 and −621) located in the promoter, were significantly related to PTB1 expression ( P <0.05, t -test) and to rice PSSRs ( P <0.05, t -test) ( Fig. 7c,d , Supplementary Data 1 ). These results revealed that the haplotype of the promoter had a role in determining the level of PTB1 expression and consequently affected the final PSSRs. Simultaneously, a superior haplotype of O. sativa , TCGT, was identified, corresponding to haplotype 12 ( Fig. 7a,b ); this enabled high PSSR selection in rice-breeding programs. PTB1 accounts for PSSR decrease under abnormal temperature Rice PSSR is affected by environmental temperature, especially during the flowering stage, and this always leads to a great loss in rice yields. Therefore, we surveyed whether PTB1 was involved in this loss of grain yield. 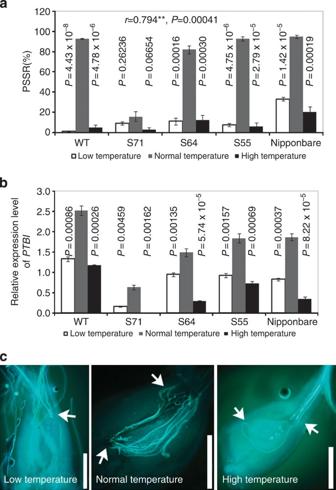Figure 8:PTB1is responsible for the PSSR decrease mediated by abnormal temperatures. (a) Variations in PSSR under the treatment temperatures. Values represent the mean±s.e.m. (n=3). WT (indica) and Nipponbare (japonica), together with three otherptb1–PTB1transgenic lines with different PSSRs, S71, S64 and S55, were treated with normal, lower and higher temperatures for 5 days. (b) Relative expression levels ofPTB1under the treated temperatures. The relative expression level of thePTB1gene in each accession was determined using q-PCR with RNA isolated from the flag leaves of each treated plant. The relative expression levels are measured as the mean±s.e.m. (n=3). EachP-value is based on a two-tailedt-test for the treatment and normal temperatures. Thervalue indicates the correlation between PSSRs and the relative expression levels ofPTB1under given conditions (P<0.01, Pearson correlation analysis). (c) PT growth of the WT at various temperatures. Arrows indicate the chalazal end of the embryo sac and the micropyle. Samples were collected for fluorescence microscopic observation at 2 h AP,n>30. Scale bars, 400 μm. The results showed that all plants PSSRs were affected by abnormal conditions, especially by high temperature ( Fig 8a , P <0.01, t -test). In accordance with the decrease in PSSR, the PTB1 expression level was dramatically downregulated under abnormal temperatures ( Fig. 8b , P <0.01, t -test), and the variations in PSSR and gene expression were significantly correlated ( Fig. 8a,b , r =0.794, P <0.01, Pearson correlation analysis). We thus infer that the environmental temperature mediated the instability of rice PSSR, which directly determines varietal adaptability, and that this may be caused by alterations in the expression of PTB1 . Figure 8: PTB1 is responsible for the PSSR decrease mediated by abnormal temperatures. ( a ) Variations in PSSR under the treatment temperatures. Values represent the mean±s.e.m. ( n =3). WT ( indica ) and Nipponbare ( japonica ), together with three other ptb1–PTB1 transgenic lines with different PSSRs, S71, S64 and S55, were treated with normal, lower and higher temperatures for 5 days. ( b ) Relative expression levels of PTB1 under the treated temperatures. The relative expression level of the PTB1 gene in each accession was determined using q-PCR with RNA isolated from the flag leaves of each treated plant. The relative expression levels are measured as the mean±s.e.m. ( n =3). Each P -value is based on a two-tailed t -test for the treatment and normal temperatures. The r value indicates the correlation between PSSRs and the relative expression levels of PTB1 under given conditions ( P <0.01, Pearson correlation analysis). ( c ) PT growth of the WT at various temperatures. Arrows indicate the chalazal end of the embryo sac and the micropyle. Samples were collected for fluorescence microscopic observation at 2 h AP, n >30. Scale bars, 400 μm. Full size image We then observed PT growth under certain conditions to further confirm our conclusions. As shown in the WT, PT growth in all treated plants was greatly affected under both higher and lower temperatures. The majority of PTs encountered sudden arrest at the sporophytic STT near the chalazal end of the embryo sac, and few or no PTs continued their journey to reach the micropyle ( Fig. 8c ); this result is similar to the results observed in the transgenic lines in which PTB1 was expressed at low or moderate levels in a ptb1 background ( Fig. 6a,b ). Although other unknown factors may also be involved in this yield-loss process, these observations demonstrate that abnormal rice PSSR is due to PT growth arrest in the STT, where the PTB1 PT growth-controlling function is inhibited due to the downregulation of PTB1 expression at higher and lower temperatures. PTB1 expression patterns To examine the temporal and spatial expression patterns of PTB1 , we generated a construct in which the β-glucuronidase ( GUS ) gene was driven by the ~1.5-kb PTB1 promoter for the transformation of rice and Arabidopsis . Histochemical staining suggested that PTB1 was differentially expressed in various rice tissues; expression was relatively weak in the root, shoot and leaf ( Fig. 9a–d ), and was strong in the stigma of the pistil and the spikelet hulls of the pre-emergence panicle ( Fig. 9e–g ). However, the expression of PTB1 in rice pollen grains was undetectable ( Fig. 9h,i ). These observations were similar to findings in transgenic Arabidopsis , where PTB1 was strongly expressed in the stigma and the upper style but barely expressed in pollen grains ( Supplementary Fig. S6 ). Q-PCR analysis further confirmed this result by showing that PTB1 was expressed preferentially in reproductive organs such as the pistil, young panicle, pre-emergence panicle and post-emergence panicle ( Fig. 9i ). The expression pattern of PTB1 corresponded well to its role in PT growth. We also generated several PTB1 – HA transgenic lines, in which the ptb1 mutant phenotypes were rescued, to localize the PTB1 protein in rice tissues; however, we failed to detect the PTB1–HA fusion protein by western blotting. 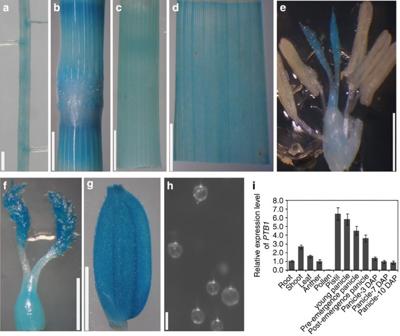Figure 9: Expression patterns ofPTB1. (a–h) GUS activity in various organs of PPTB1-GUS-transformed rice plants. (a) Growing root, (b) stem node, (c) stem internode, (d) leaf, (e) floret, (f) pistil, (g) shell of unpollinated spikelet and (h) pollen grains. (i) RelativePTB1transcript levels of several tissues detected by q-PCR analysis. DAP, days after pollination. Values represent the mean±s.e.m. (n=3). Scale bars, 400 μm in (a), 3 mm in (b) and (c), 1 cm in (d), 1 mm in (e) and (f), 4 mm in (g) and 50 μm in (h). Figure 9: Expression patterns of PTB1 . ( a – h ) GUS activity in various organs of P PTB1 - GUS -transformed rice plants. ( a ) Growing root, ( b ) stem node, ( c ) stem internode, ( d ) leaf, ( e ) floret, ( f ) pistil, ( g ) shell of unpollinated spikelet and ( h ) pollen grains. ( i ) Relative PTB1 transcript levels of several tissues detected by q-PCR analysis. DAP, days after pollination. Values represent the mean±s.e.m. ( n =3). Scale bars, 400 μm in ( a ), 3 mm in ( b ) and ( c ), 1 cm in ( d ), 1 mm in ( e ) and ( f ), 4 mm in ( g ) and 50 μm in ( h ). Full size image To investigate the subcellular localization of PTB1, we constructed a PTB1 – YFP (yellow fluorescent protein) fusion construct whose expression was driven by the CaMV 35S promoter. Interestingly, transient expression in rice protoplast cells showed that PTB1–YFP localized preferentially to the cytoplasm and was weakly expressed on the membrane ( Supplementary Fig. S7 ), although the PTB1 protein was predicted to contain four transmembrane segments. It will be worth investigating the localization of PTB1 by generating transgenic rice lines expressing biologically functional PTB1–YFP fusion protein in future studies. PTB1 has E3 ubiquitin ligase activity The PTB1 gene contained 10 exons and encoded a putative protein with 387 amino acids. An analysis of the predicted sequence revealed four transmembrane regions at AA 12–146 and a conserved RING finger domain (belonging to the canonical RING-H2 type) [30] , [31] , [32] at AA 234–274 ( Supplementary Fig. S3 ). A phylogenetic analysis of PTB1 homologues showed that two major classes, the monocotyledonous clade and the dicotyledonous clade, were constructed; this finding might suggest a possible conserved role for PTB1 in related species ( Supplementary Fig. S8 ). RING-type proteins are widely present in various organisms and have been verified to function as E3 ubiquitin ligases [4] , [33] , [34] , [35] . We cloned and expressed the intact RING functional region of PTB1 in Escherichia coli and then used the GST-tagged GST-RING to verify its activity in vitro using Brassica BnTR1 (ref. 36 ) as a positive control. In the presence of ubiquitin, E1 and E2 (UbcH5b), BnTR1 or GST-RING could carry out self-ubiquitination, whereas in the absence of any of the E1, E2 or E3 enzymes, no clear protein ubiquitination was detected ( Fig. 10a ). These results demonstrate that PTB1 possesses intrinsic E3 ligase activity. 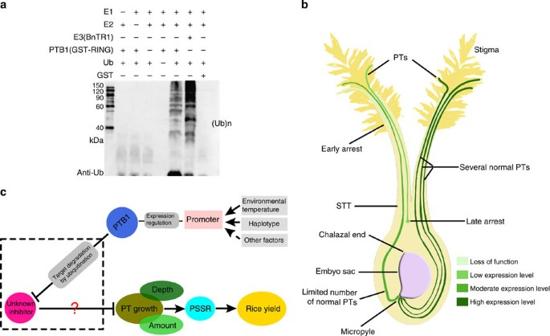Figure 10: Ubiquitination analysis and a summary of PTB1 function. (a) Ubiquitination analysis of PTB1 (GST-RING). BnTR1 and PTB1 (GST-RING) fusion proteins were assayed for E3 activity in the presence of E1, E2 and ubiquitin. (b) A sketch illustrating that the expression level ofPTB1positively regulates PT growth in rice reproductive tract.PTB1function loss caused early arrests of PT growth, and a lower expression level caused late arrests. A moderate expression level also led to late arrests, although some PTs reached the micropyle. However, a higher expression level generated several normally growing PTs that resulted in fertilization. (c) A proposed model for the role of PTB1 in the regulation of rice PSSR and yield. The steps within the box marked using a black dotted line are currently unknown. Figure 10: Ubiquitination analysis and a summary of PTB1 function. ( a ) Ubiquitination analysis of PTB1 (GST-RING). BnTR1 and PTB1 (GST-RING) fusion proteins were assayed for E3 activity in the presence of E1, E2 and ubiquitin. ( b ) A sketch illustrating that the expression level of PTB1 positively regulates PT growth in rice reproductive tract. PTB1 function loss caused early arrests of PT growth, and a lower expression level caused late arrests. A moderate expression level also led to late arrests, although some PTs reached the micropyle. However, a higher expression level generated several normally growing PTs that resulted in fertilization. ( c ) A proposed model for the role of PTB1 in the regulation of rice PSSR and yield. The steps within the box marked using a black dotted line are currently unknown. Full size image To obtain clues into the PT-controlling mechanism of PTB1 , we surveyed the expression levels of several putative rice homologues that are involved in female sterility, PT growth or callose synthesis and metabolism ( Supplementary Table S5 ). In total, 5 out of 32 surveyed rice genes were confirmed to be downregulated in ptb1 ( Supplementary Fig. S9 , P <0.01, t -test). Interestingly, four of these five genes were putative homologues of Brassica rapa S locus glycoproteins ( SLG ) [37] , [38] , [39] , which suggested that the role of PTB1 in rice PT growth might relate to self-incompatibility, although the latter remains unknown in rice. The remaining gene was a putative homologue of Arabidopsis UNE15 (ref. 40 ), a gene that appears to be involved in PT attraction. However, none of these genes has been functionally characterized. In this study, we report the cloning of PTB1 and its role in regulating rice PSSR by controlling PT growth. PTB1 expression is significantly correlated with rice PSSR both in transgenic plants and in natural populations. We also show that PTB1 is strongly expressed in the stigma and style and that it encodes a RING-type E3 ubiquitin ligase. Additionally, the PTB1 locus has been shown to present a potential signature of domestication, and the promoter haplotype contributes to the variation in PTB1 expression. Our data therefore reveal a key factor for PT growth and an important regulator of rice PSSR. Although abnormalities of PTs within the rice pistil result in a spectrum of growth phenotypes depending on the PTB1 expression level, none are observed to exhibit the classic defects in PT micropyle guidance [16] , [41] ( Figs 2 and 6b,d ) that are generally believed to be controlled by cues emitted from the female gametophyte [19] , [20] , [21] . This finding is consistent with the result that the mature embryo sac of the mutant is morphologically normal ( Supplementary Fig. S1 ) and that PTB1 is prevailingly expressed in the rice stigma and style ( Fig. 9 , Supplementary Fig. S6 ). These results indicate that PTB1 has a sporophytic role during the long-distance navigation of PTs toward the female gametophyte in rice and that it is not involved in the last step of gametophyte guidance. Genetic evidence provided by both PT growth ( Fig. 3 ) and the final seed setting ( Supplementary Table S1 ) of the reciprocal crossing has demonstrated that the PT growth arrest of the mutant is caused by a maternal defect and that the mutation does not affect the function of the male gametophyte; therefore, we conclude that PTB1 is a key maternal sporophytic factor of PT growth in rice. PTB1 has pleiotropic effects on PT growth control. First, it has a decisive role in entering and early growth of the STT. As we discovered for the ptb1 (loss of function) mutant, most PTs are detained in the lower end of the stigma or blocked during the early stages of STT navigation ( Fig. 2 ). Second, PTB1 functions during the later navigation of PTs in the STT because a lower level of PTB1 expression leads to different numbers of PTs growing in this process, as observed in the transgenic plants with lower PSSRs ( Fig. 6a,b ). Third, PTB1 promotes growth from the chalazal end of the sporophytic STT to the micropyle because a moderate expression of PTB1 leads to the growth of few PTs in this female location, as observed in the transgenic plants with moderate PSSRs ( Fig. 6a,b ). Finally, PTB1 functions as a promoting agent based on the observation that a higher expression of this gene encourages more PTs to complete their full journey, as observed in the transgenic plants with higher PSSRs ( Fig. 6a,b ). These observations suggest that PTB1 has a role in promoting the amount and depth of growth of PTs in the rice reproductive tract, indicating that the level of PTB1 expression positively regulates PT growth in a dose-dependent manner ( Fig. 10b ). However, the PTB1 protein itself might not act as a direct PT promoter reagent, considering its role as an E3 ubiquitin ligase ( Fig. 10a ). Thus, we propose that PTB1 recruits its substrate (an unknown inhibitor of PT growth) for target degradation, thereby promoting PT growth by controlling the amount and depth of growth of PTs and, subsequently, positively affecting rice PSSR and ultimately improving grain yields ( Fig. 10c ). Simultaneously, the environmental temperature ( Fig. 8 ) and the promoter haplotype ( Fig. 7c,d ) have roles in regulating the expression level of PTB1 , thereby also modulating rice PSSR. The identification and characterization of the substrate-binding domain of PTB1 and the PTB1 target substrate will be challenging but should prove interesting for uncovering the mechanism by which the ubiquitination system contributes to the regulation of PT growth, PSSR and the resultant grain yields in plants. Possibly because they are affected by many environmental factors, no genes regulating PSSR have been functionally reported to our knowledge, and the mechanism involved remains currently unknown in rice. PSSR, although a yield-related trait, is fundamentally determined by the reproduction-related factors, which suggests a shortcut that might enable us to dissect the complex yield trait, PSSR, by investigating genes that are related to reproduction. As pollen grains are always present in surplus during plant reproduction, genes related to male function may be less important than maternal factors (such as genes that control female gametophyte development or that mediate the maternal influence on pollination) in determining the final PSSR ( Fig. 6d,e ). In the present study, we have demonstrated that a maternal PT growth-controlling gene has an essential role in rice PSSR regulation, which might suggest that other maternal factors also participate in this process, at least for those factors that are involved in the PTB1 regulating pathway. Thus, our findings provide an initial step toward dissecting the mechanism that underlies the regulation of PSSR and grain yield in plants. In addition, we found that the environmental temperature-mediated instability of rice PSSR is caused by the downregulation of PTB1 ( Fig. 8 ), which explains why rice yield loss occurs under abnormal temperatures; this finding may benefit our understanding of the geographic distribution and adaptability of rice varieties. We also show that higher expression levels of PTB1 have a tendency to improve rice PSSR ( Supplementary Fig. S5 ); this finding suggests new strategies for improving rice yields. Crop domestication is the genetic modification of a wild species to generate a new form of a crop altered to meet human needs [42] . Recently, several rice domestication-related traits such as grain shattering [43] , [44] , prostrate growth habit [45] , [46] , pericarp colour [47] , grain size [3] , [4] , [5] and inflorescence architecture [48] , [49] have been well characterized. From a yield improvement viewpoint, it is understandable that the transition from a lower to a higher PSSR is a critical event for rice domestication. The PTB1 haplotypes of cultivated rice, especially of indica varieties, are significantly limited compared with that of O. rufipogon , suggesting that strong selection occurred during rice domestication ( Fig. 7a,b ). This result was further supported by recent independent work [29] carried out by re-sequencing 446 O. rufipogon accessions and 1,083 cultivated varieties, in which a 400-kb selective sweep region around the PTB1 gene was identified in an indica population. Considering that the haplotype of the promoter has a role in determining the expression level of PTB1 ( Fig. 7c,d ), we infer that the causal mutation (haplotype) of the PTB1 promoter was the target for artificial selection by ancient humans, which led to an increase in grain yield to meet human needs during rice domestication. Plant materials and growing conditions The ptb1 mutant used here was obtained from a spontaneous mutation in an indica cultivar, X3107. Several other rice cultivars used in the reciprocal crossing and genetic analysis are listed in Supplementary Tables S1 and S2 . From these cultivars, a mapping population of 2,382 F 2 mutant plants was generated from crosses between ptb1 and Gui630. Other rice lines used for natural variation analysis and haplotype analysis are listed in Supplementary Table S4 and Supplementary Data 1 . All plants were planted in the experimental field of the Rice Research Institute, Sichuan Agricultural University, Wenjiang. Phenotypic characterization Mature embryo sacs ( n >50) were examined using the WE-CLSM method [25] . PT growth behaviours were observed using an aniline blue staining method. More than 30 pollinated pistils for the mutant and WT were first collected at each of 5 min, 10 min, 20 min, 30 min, 45 min, 60 min, 120 min, 12 h and 48 h AP and fixed in Carnoy’s fixing reagent (30% chloroform, 10% acetic acid and 57% ethanol). The samples were then washed with water, incubated in 10 mol l −1 NaOH for 6–10 min at 56 °C and stained in 0.1% aniline blue solution for 8–12 h for fluorescent observation. For STT observation, the female reproductive tract was first observed using a modified WE-CLSM method [25] in which eosin B was substituted with propidium iodide for staining; the sample was then further analysed using Alcian blue staining of paraffin sections of pistils at the flowering stage according to Crawford et al . [27] Mapping and cloning of PTB1 PTB1 was mapped primarily with simple sequence repeat markers using 100 F 2 mutant plants. The PTB1 locus was further narrowed down to a 72-kb region between markers RL33 and RD19 using 2,382 F 2 mutant plants and newly developed molecular markers. Sequence deletion in the mutant was confirmed using PCR with the primer set D PTB1 and using RT–PCR with CD PTB1 . The full-length cDNA of the candidate gene was then amplified from the first-strand cDNA of WT plants using the primer set C PTB1 , and the promoter regions upstream of the ATG start codon were amplified directly from the genomic DNA of WT plants using P PTB1 . All primers used for the map-based cloning and functional analysis of PTB1 are listed in Supplementary Table S6 . Expression analysis Total RNA was extracted from various rice tissues using TRIzol reagent (Invitrogen) and reverse transcribed using the TransScript One-Step gDNA Removal and cDNA Synthesis SuperMix kit (TransGen); RT–PCR was then performed according to the manufacturer’s instructions. q-PCR was carried out in a total volume of 10 μl containing 0.3 μl of reverse-transcribed product, 0.08 mM gene-specific primers and 5.0 μl of SsoAdvancedTM SYBR Green Supermix (Bio-Rad) using a Bio-Rad CFX96 Real-Time PCR System according to the manufacturer’s instructions. Measurements were obtained using the relative quantification method [50] . The rice Actin gene was used as the internal control. Each measurement was determined for at least two biological samples and using three replicates for each sample. Construction and transgenic analysis We first generated an overexpression construct, pHB– PTB1 –OVE, by inserting full-length PTB1 cDNA from the WT into the plant binary vector pHB [28] . We then generated the complementary construct pHB– PTB1 –COM by substituting the 2 × CaMV 35S promoter of pHB– PTB1 –OVE with the native PTB1 promoter. For the tissue localization of PTB1 , a P PTB1 - GUS construct in which the GUS gene was driven by the PTB1 promoter was generated by substituting the 35S promoter of GUS with the native PTB1 promoter on pCMBIYA1300. All constructs were introduced into the Agrobacterium tumefaciens strain EHA105; pHB– PTB1 –OVE and P PTB1 - GUS were transferred into an indica variety (kasalath) and Arabidopsis columbia. As the mutant was sterile and could not generate seeds for callus induction, the complementary construct pHB– PTB1 –COM was introduced into the young panicle-originated callus of the ptb1 mutant. Genetic transformation was performed according to Hiei et al . [51] To investigate the subcellular localization of PTB1, we constructed a pA7– PTB1 – YFP (yellow fluorescent protein) fusion construct whose expression was driven by the CaMV 35S promoter for transiently transforming the rice protoplast. E3 ubiquitin ligase activity assay Although several expression systems were attempted, we failed to express the full PTB1 protein in vitro . Therefore, we selected an eclectic method by cloning the intact RING functional region of PTB1 and fusing it to the 3′ end of GST. The fusion protein was then prepared for ubiquitination analysis according to the manufacturer’s protocol. Assays for in vitro ubiquitination were carried out according to the protocols of Song et al . [4] and Liu et al . [36] Brassica napus E3 ubiquitin ligase BnTR1 (ref. 36 ) was used as a positive control, and GST was used as a negative control. Ubiquitinated proteins were detected by protein blot analysis using an ubiquitin antibody (Cell Signaling Technology, 1/1,000( v / v )). Temperature treatment To simulate the influence of natural abnormal weather on rice PSSR, the normal temperature was set based on field conditions; the average temperature was ~29 °C within a range from 23–33 °C. A higher temperature was obtained using a plastic-covered chamber in the field (the average temperature was 37 °C within a range from 25–41 °C), and a lower temperature was achieved in a greenhouse (the temperature was ~19 °C within a range from 15–23 °C). At the beginning of the heading time, rice plants were transplanted into the lower, normal and higher temperature conditions for 5 days of treatment. Flag leaf samples were collected immediately after each treatment, and the PSSRs for each line were recorded using corresponding panicles. At least 30 pollinated pistil samples of the treated lines were collected at 2 h AP for the fluorescent microscopic observation of PT growth. Accession codes : The PTB1 sequence has been deposited in the GenBank nucleotide database under the accession code KC425226 . How to cite this article: Li, S. et al . Natural variation in PTB1 regulates rice seed setting rate by controlling pollen tube growth. Nat. Commun. 4:2793 doi: 10.1038/ncomms3793 (2013).